Control of lung vascular permeability and endotoxin-induced pulmonary oedema by changes in extracellular matrix mechanics Increased vascular permeability contributes to many diseases, including acute respiratory distress syndrome, cancer and inflammation. Most past work on vascular barrier function has focused on soluble regulators, such as tumour-necrosis factor-α. Here we show that lung vascular permeability is controlled mechanically by changes in extracellular matrix structure. Our studies reveal that pulmonary vascular leakage can be increased by altering extracellular matrix compliance in vitro and by manipulating lysyl oxidase-mediated collagen crosslinking in vivo . Either decreasing or increasing extracellular matrix stiffness relative to normal levels disrupts junctional integrity and increases vascular leakage. Importantly, endotoxin-induced increases of vascular permeability are accompanied by concomitant increases in extracellular matrix rigidity and lysyl oxidase activity, which can be prevented by inhibiting lysyl oxidase activity. The identification of lysyl oxidase and the extracellular matrix as critical regulators of lung vascular leakage might lead to the development of new therapeutic approaches for the treatment of pulmonary oedema and other diseases caused by abnormal vascular permeability. Vascular permeability is tightly regulated during blood vessel development and it is indispensable for normal organ function throughout adult life [1] . Many life-threatening pathological conditions, including acute respiratory distress syndrome (ARDS), atherosclerosis, cancer and organ failure are caused or complicated by compromised vascular barrier function [1] , [2] , [3] , [4] . In ARDS—a devastating pulmonary complication that often occurs with sepsis caused by systemic infection—excess fluid leaks out of the lung capillaries and fills the adjacent alveolar air spaces causing pulmonary oedema [5] ; this fluid impairs gas exchange across the alveolar membrane, decreases lung compliance and severely compromises respiratory function. ARDS occurs in almost half of severe sepsis cases in human patients and combination of sepsis and ARDS is associated with a mortality of 60% ( [6] ). Despite a great amount of effort in this area, currently there is no specific clinical therapy for ARDS or any other condition caused by abnormal vascular permeability. Work on control of vascular permeability has focused on the role of critical soluble inflammatory regulators of endothelial barrier function, such as vascular endothelial growth factor (VEGF) [4] , [7] , tumour-necrosis factor (TNF)-α ( [8] ), transforming growth factor-β ( [9] ), and interleukin (IL)2 ( [10] ), among others. Indeed, the levels of these chemical factors are elevated in lung epithelial lining fluid collected from patients with early phase of ARDS, and they seem to have a key role in the pathogenesis of this disease [11] , [12] . The present study was initiated based on the recent finding that VEGF-induced angiogenesis can be regulated by changes in the mechanical properties (for example, physical compliance) of the extracellular matrix (ECM), which also has a central role in control of stem cell fate switching and tissue development, as well as cancer formation [13] , [14] , [15] , [16] . Changes in ECM structure can normalize tumour microvessels [17] , which are known to be hyperpermeable [4] , and bleomycin-induced pulmonary fibrosis is accompanied by increases in both lung stiffness [18] and vascular permeability [19] . Stiffening of ECM within the vascular intima also promotes endothelial cell permeability during atherosclerosis progression [20] . Taken together, these observations raised the intriguing possibility that physical changes in ECM mechanics might actively regulate lung vascular permeability. Here we show that ECM structure and mechanics have key roles in control of vascular permeability and endotoxin-induced pulmonary oedema. The ECM controls endothelial cell–cell junction formation Various diseases, such as cancer and fibrosis, that are accompanied by abnormal vascular permeability also exhibit altered tissue mechanics (for example, increased stiffness) [4] , [13] , [18] , [19] , [20] . We, therefore, explored whether changes in mechanical interactions between cells and ECM might regulate vascular permeability by culturing lung human microvascular endothelial (L-HMVE) cells on fibronectin-coated polyacrylamide gels with different stiffness (Young’s moduli of 150–35,000 Pa) ( [15] ). When cells were cultured on substrates with an intermediate stiffness (4,000 Pa), they flattened and exhibited well-developed cell–cell adhesions, whereas when the same cells were grown on more flexible substrates (150 Pa), they appeared round, vascular endothelial (VE)-cadherin-containing cell–cell junctions became disrupted, and this was associated with increased VE-cadherin staining in the cytoplasm ( Fig. 1a ). Interestingly, cell–cell adherens junctions also were disrupted in cells cultured on abnormally rigid gels (35, 000 Pa) ( Fig. 1a ), suggesting that a normal level of intermediate ECM stiffness is necessary to maintain optimal cell–cell junctional integrity. This effect appeared to be linked to ECM mechanics per se in that a similar trend was also observed in the L-HMVE cells cultured on different stiffness polyacrylamide gels coated with type I or type IV collagen ( Supplementary Figs S1a,b ). In addition, when we stained cells with the tight junction protein, ZO1, we detected similar mechanical control of tight junction integrity by varying ECM elasticity ( Fig. 1c ). Thus, ECM stiffness per se appears to be a critical determinant of pulmonary endothelial barrier function in vitro . Moreover, when endothelial cell–cell junctional integrity was measured by quantifying transendothelial electrical resistance (TEER), cells grown on the gels with intermediate stiffness (4, 000 Pa) consistently displayed the highest TEER, indicating that an appropriate (intermediate) ECM stiffness is also necessary to maintain normal integrity of cell–cell junctions and associated vascular permeability barrier function in vitro ( Fig. 1d ). 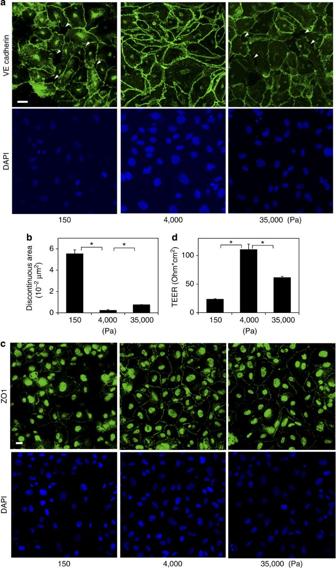Figure 1: Matrix elasticity controls the integrity of endothelial cell–cell junction. (a) Immunofluorescence micrographs showing cell–cell junction structure by VE-cadherin staining and nuclei by DAPI staining in L-HMVE cells on gels of different elasticity coated with fibronectin (bar, 5 μm). Arrowheads show the region where cell–cell junctions are disrupted. (b) Graph showing the quantitation of the total discontinuous area of at least 10 fields (*,P<0.01, unpairedT-test). (c) Immunofluorescence micrographs showing tight junction structure by ZO1 staining and nuclei by DAPI staining in L-HMVE cells on gels of different elasticity coated with fibronectin (FN) (bar, 5 μm). (d) Graph showing endothelial cell–cell junctional integrity measured by TEER in the L-HMVE cells cultured on gels with different elasticity (n=8, *,P<0.05, unpairedT-test). All error bars are s.e.m. Figure 1: Matrix elasticity controls the integrity of endothelial cell–cell junction. ( a ) Immunofluorescence micrographs showing cell–cell junction structure by VE-cadherin staining and nuclei by DAPI staining in L-HMVE cells on gels of different elasticity coated with fibronectin (bar, 5 μm). Arrowheads show the region where cell–cell junctions are disrupted. ( b ) Graph showing the quantitation of the total discontinuous area of at least 10 fields (*, P <0.01, unpaired T -test). ( c ) Immunofluorescence micrographs showing tight junction structure by ZO1 staining and nuclei by DAPI staining in L-HMVE cells on gels of different elasticity coated with fibronectin (FN) (bar, 5 μm). ( d ) Graph showing endothelial cell–cell junctional integrity measured by TEER in the L-HMVE cells cultured on gels with different elasticity ( n =8, *, P <0.05, unpaired T -test). All error bars are s.e.m. Full size image Lysyl oxidase inhibition increases pulmonary vascular leakage in vivo To determine whether changes of ECM stiffness regulate pulmonary vascular permeability in vivo , we inhibited collagen and elastin crosslinking in mice by treating them with the lysyl oxidase (LOX) activity inhibitor, beta-aminopropionitrile (BAPN) [21] , [22] , and in separate mice, we increased ECM crosslinking (and hence, rigidity) by injecting DNA encoding the LOX enzyme [3] , [23] , [24] . Treatment of mice with BAPN (which has been previously shown to disrupt collagen fibre structure in mammary tumors [13] ) for 2 weeks resulted in a 25% decrease in LOX activity measured in blood samples ( Fig. 2 ). To directly examine whether LOX inhibition altered ECM structure, whole lungs were decellularized by perfusing mice with detergent-containing buffer ( Supplementary Fig. S2a ). The detergent-extracted lungs extracted all of the cellular contents from the lung as detected by removal of 4',6-diamidino-2-phenylindole (DAPI) staining ( Supplementary Fig. S2b ), but retained normal microarchitecture [25] , [26] , including ECMs delineating large vessels surrounded by alveoli, alveolar septae, the characteristic spongy matrix of the lung ( Fig. 2a , top) and fine ECM fibrils containing collagen I, III, IV, VI, major collagens in the lung, when analysed by immunofluorescence microscopy ( Fig. 2a and Supplementary Fig. S2c ). In contrast, BAPN-treated lungs lost the fine network of collagen I, III, IV, VI-containing fibrils, and the normally well-defined borders of alveolar structures were disrupted ( Fig. 2a and Supplementary Fig. S2c ). However, BAPN treatment did not significantly alter messenger RNA (mRNA) expression of these collagens, and the proportion of each collagen type was similar to that exhibited by control lungs ( P >0.05, unpaired T -test). We confirmed these results by quantitating 4-hydroxyproline levels as a measure of the amount of collagen present in the tissue [27] . BAPN treatment did not significantly alter lung hydroxyproline levels, and there was no change in the hydroxyproline levels in serum ( P >0.05, unpaired T -test), which are commonly elevated with increased collagen turnover [28] . These results indicate that the short-term (2 week) BAPN treatment we utilized did not significantly alter the production or degradation of collagen in the lung. 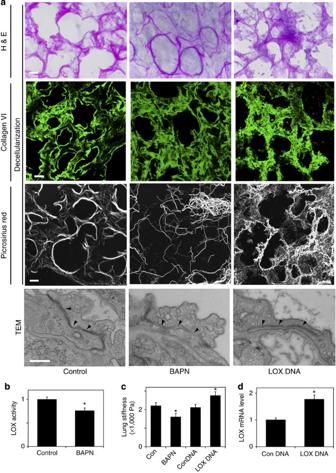Figure 2: LOX regulates ECM structure and cell–cell junctional integrity in the lungin vivo. (a) ECM structure in the control versus BAPN or LOX DNA-treated mouse lungs.top, light (Haematoxylin and eosin-stained) micrographs showing ECM structure of decellularized lung treated with BAPN or LOX DNA (bar, 3 μm).2nd, Immunofluorescence micrographs showing Collagen VI distribution in the control versus BAPN or LOX DNA-treated decellularized lung (bar, 4 μm).3rd, birefringence (Picrosirius Red-stained) micrographs showing collagen structure of decellularized lung treated with BAPN or LOX DNA (bar, 3 μm).Bottom, TEM images showing endothelial cell–cell junctional integrity in the lung treated with BAPN or LOX DNA (bar, 500 nm). Arrowheads show the region of cell–cell junctions. (b) Graph showing LOX activity in blood in mice treated with LOX inhibitor BAPN (n=10, *P<0.01, unpairedT-test). (c) Graph showing lung stiffness measured by the tensile loading assay in the mice treated with BAPN, control DNA (con DNA, vector only) or LOX DNA (n=10, *,P<0.05, unpairedT-test). (d) mRNA levels of LOX in mouse lungs treated with control DNA (con DNA, vector only) or LOX DNA (n=9, *,P<0.05, unpairedT-test). All error bars are s.e.m. Figure 2: LOX regulates ECM structure and cell–cell junctional integrity in the lung in vivo. ( a ) ECM structure in the control versus BAPN or LOX DNA-treated mouse lungs. top , light (Haematoxylin and eosin-stained) micrographs showing ECM structure of decellularized lung treated with BAPN or LOX DNA (bar, 3 μm). 2nd , Immunofluorescence micrographs showing Collagen VI distribution in the control versus BAPN or LOX DNA-treated decellularized lung (bar, 4 μm). 3rd , birefringence (Picrosirius Red-stained) micrographs showing collagen structure of decellularized lung treated with BAPN or LOX DNA (bar, 3 μm). Bottom , TEM images showing endothelial cell–cell junctional integrity in the lung treated with BAPN or LOX DNA (bar, 500 nm). Arrowheads show the region of cell–cell junctions. ( b ) Graph showing LOX activity in blood in mice treated with LOX inhibitor BAPN ( n =10, * P <0.01, unpaired T -test). ( c ) Graph showing lung stiffness measured by the tensile loading assay in the mice treated with BAPN, control DNA (con DNA, vector only) or LOX DNA ( n =10, *, P <0.05, unpaired T -test). ( d ) mRNA levels of LOX in mouse lungs treated with control DNA (con DNA, vector only) or LOX DNA ( n =9, *, P <0.05, unpaired T -test). All error bars are s.e.m. Full size image To more carefully analyse changes in collagen structure, we performed picrosirius red staining, which detects fibrillar collagen (types I—V) ( [29] ) within decellularized lung sections, and examined collagen fibre microarchitecture using birefringence microscopy [29] , [30] . In control lungs, collagen fibres aligned with the alveolar septae, whereas they appeared to be more randomly distributed in BAPN-treated lungs ( Fig. 2a ). Thus, continuous ECM crosslinking appears to be required to maintain normal alveolar architecture in whole lung. The junctional integrity of the pulmonary endothelium was also analysed in control and BAPN-treated mice using transmission electron microscopy (TEM). Junctions between pulmonary endothelial cells were tight and characterized by closely apposed membranes in randomly sampled regions of lung from untreated mice. In contrast, cell–cell junctions appeared to be disrupted with increased space appearing between adjacent cell membranes in lungs from BAPN-treated mice ( Fig. 2a ). When we measured lung mechanics using a tensile loading assay [31] , [32] , the stiffness (Young’s modulus) of BAPN-treated lung was found to decrease by 40% compared with controls ( Fig. 2c ), as expected from treatment with this ECM crosslinking inhibitor. Importantly, BAPN treatment also increased lung vascular permeability, as detected by leakage of fluorescently labelled low molecular weight (MW) dextran ( Fig. 3a ) or Evans Blue dye; leakage was >60% higher than in control non-treated lungs ( Fig. 3b and Supplementary Fig. S3a ). In addition, BAPN treatment increased inflammatory cells in the bronchoalveolar lavage (BAL) fluid by ~2-fold, and this was mainly attributable to an increase in neutrophils and monocytes ( Fig. 3d ). However, BAPN treatment did not significantly increase the levels of the key inflammatory mediators, IL-1 or TNFα in the lung when analysed by enzyme-linked immunosorbent assay (ELISA) ( Supplementary Fig. S3b ). These findings are consistent with BAPN increasing lung vascular permeability by changing ECM structure and mechanics, rather than by inducing secondary inflammatory effects. The finding that BAPN treatment also did not produce detectable changes in lung cell proliferation or apoptosis in vivo (not shown), further suggests that the observed effects of BAPN on vascular permeability are due to direct disruption of junction integrity, and not to cell death. 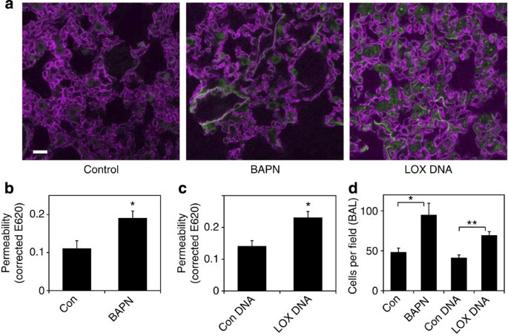Figure 3: LOX regulates lung vascular permeabilityin vivo. (a) Immunofluorescence micrographs showing low MW fluorescently labelled dextran leakage (green) and blood vessel formation (CD31 staining; magenta) in BAPN- or LOX DNA-treated mouse lung (bar, 10 μm). (b) Vascular permeability in mouse lungs treated with BAPN. Vascular permeability is detected by Evans Blue dye leakage in the lungs treated with BAPN and extracted dye contents are quantified by measuring at 620 nm (n=9, *,P<0.05, unpairedT-test). (c) Vascular permeability in mouse lungs treated with control DNA (con DNA) or LOX DNA. Graph showing vascular permeability detected by Evans Blue dye leakage in the lungs overexpressed with LOX DNA (n=9, *,P<0.05, unpairedT-test). (d) Graph showing the total inflammatory cell count in BAL fluid from the lungs treated with BAPN, control DNA (con DNA) or LOX DNA detected by Wright-Giemsa staining (n=8, *,P<0.01, **,P<0.05, unpairedT-test). All error bars are s.e.m. Figure 3: LOX regulates lung vascular permeability in vivo . ( a ) Immunofluorescence micrographs showing low MW fluorescently labelled dextran leakage (green) and blood vessel formation (CD31 staining; magenta) in BAPN- or LOX DNA-treated mouse lung (bar, 10 μm). ( b ) Vascular permeability in mouse lungs treated with BAPN. Vascular permeability is detected by Evans Blue dye leakage in the lungs treated with BAPN and extracted dye contents are quantified by measuring at 620 nm ( n =9, *, P <0.05, unpaired T -test). ( c ) Vascular permeability in mouse lungs treated with control DNA (con DNA) or LOX DNA. Graph showing vascular permeability detected by Evans Blue dye leakage in the lungs overexpressed with LOX DNA ( n =9, *, P <0.05, unpaired T -test). ( d ) Graph showing the total inflammatory cell count in BAL fluid from the lungs treated with BAPN, control DNA (con DNA) or LOX DNA detected by Wright-Giemsa staining ( n =8, *, P <0.01, **, P <0.05, unpaired T -test). All error bars are s.e.m. Full size image LOX overexpression increases vascular leakage in the lung Stimulation of ECM crosslinking through overexpression of LOX DNA by retro-orbital injection, which increased LOX mRNA and protein expression in the lung ( Fig. 2d , Supplementary Fig. S2d ), but not in other organs, such as the kidney (not shown), increased lung stiffness ( Fig. 2c ) and pulmonary vascular permeability ( Fig. 3a ) by 1.5-fold compared with lungs treated with control DNA. LOX DNA overexpression also increased the total number of inflammatory cells in the BAL fluid by ~1.5-fold ( Fig. 3d ). While retro-orbital injection of LOX DNA increased LOX expression in the lung ( Fig. 2d and Supplementary Fig. S2d ), it did not change protein levels of the other major LOXL isoform, LOXL1 ( Supplementary Fig. S2d ); LOXL2 levels were not detectable in healthy mouse lungs, as reported previously [33] . Thus, the effects of LOX DNA on lung vascular permeability appear to be specifically due to the change in expression of the LOX isoform. In addition, LOX DNA overexpression resulted in disruption of fine collagen fibril structures ( Fig. 2a and Supplementary Fig. S2c ) when compared with lungs treated with control DNA where the ECM structures appeared well-organized ( Supplementary Fig. S2e ), but it did not produce any significant effect ( P >0.05) on mRNA expression of collagen types I, III, IV or VI. Importantly, LOX DNA overexpression also increased opening of junctions between pulmonary endothelial cells ( Fig. 2a ). One potential caveat in these studies is that BAPN can block other amine oxidases and it can suppress the activity of LOXL1-4 isoforms in addition to inhibiting LOX [33] , [34] , [35] . To more directly modify this pathway, we treated mice with a LOX-specific antibody (Ab) [13] , [36] , which has been previously shown to inhibit LOX activity and disrupt collagen organization in vitro and in vivo [13] , [36] , [37] . Treatment with this LOX inhibitory Ab resulted in a 60% decrease in LOX activity measured in blood samples and it decreased lung stiffness by 30% compared with control IgG-treated lungs when measured using the tensile loading assay ( Supplementary Fig. S4a ). We also treated mice with LOX-specific short interfering RNA (siRNA) for 1 week [13] , which resulted in a 60% decrease in LOX activity measured in blood samples ( Supplementary Fig. S4c ) and specifically decreased LOX expression in the lung ( Supplementary Fig. S2d ). Treatment with LOX-specific siRNA for 1 week [13] also decreased lung stiffness by 30% compared with control siRNA-treated lungs ( Supplementary Fig. S4c ). In addition, LOX Ab or LOX siRNA treatment disrupted normal collagen fibre alignment surrounding alveolar septae ( Supplementary Fig. S4b,d ), and increased vascular permeability by 4- and 2.5-fold, respectively ( Supplementary Fig. S4b,d ). Thus, the activity of the LOX isoform itself appears to control normal alveolar architecture and vascular permeability in whole mouse lung. Mechanical control of vascular leakage in a mouse ARDS model To determine the potential clinical relevance of this pathway, we exposed whole lung of living adult mice to the endotoxin, lipopolysaccharide (LPS), which contributes to development of pulmonary oedema and ARDS in humans with sepsis [3] . As sepsis is one of the leading causes of ARDS, systemic LPS treatment is a widely accepted physiological animal model for sepsis-induced ARDS [3] , [38] . LPS treatment for 2 days increased lung vascular permeability by fourfold compared with control untreated mice ( Fig. 4a ). Interestingly, when we measured the material properties of mouse lungs under tensile loading, LPS-treated lungs also were 35% stiffer than control non-treated lungs ( Fig. 4c ), and they consistently exhibited LOX mRNA levels and activities that were 2-fold and 1.8-fold higher than those observed in control lungs, respectively ( Fig. 4d ). LPS treatment also increased LOX and LOXL1 protein levels, but had no effect on LOXL2 protein levels ( Fig. 4f and Supplementary Fig. S5a ). In addition, we found that collagen VI-positive ECM fibres were disrupted by LPS when analysed in decellularized lungs ( Fig. 5a and Supplementary Fig. S5b ), a pattern that was similar to that seen in lungs treated with LOX DNA ( Fig. 2a and Supplementary Fig. S2c ), and BAPN treatment prevented this disruption ( Fig. 5a ). Importantly, BAPN also prevented the increase of vascular permeability induced by LPS ( Fig. 5b and Supplementary Fig. S5c ). In addition, we confirmed that this effect is caused by changes in activity of the LOX isoform by showing that the increase of vascular permeability induced by LPS was restored by treatment with either LOX-specific siRNA or with LOX inhibitory Ab ( Fig. 5c ). These findings suggest that endotoxin-induced increases in vascular permeability during development of pulmonary oedema are mediated by changes in ECM structure and mechanics. 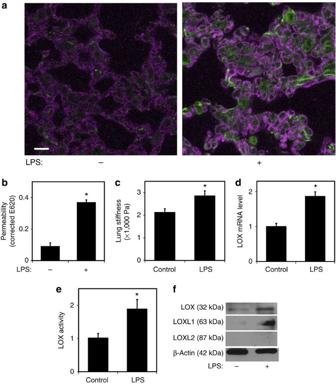Figure 4: Lung vascular permeability in endotoxin-induced lung injuryin vivo. (a) Immunofluorescence micrographs showing low MW fluorescently labelled dextran leakage (green) and blood vessel formation (CD31 staining; magenta) in LPS-treated mouse lung (for 2 days, bar, 10 μm). (b) Vascular permeability detected by Evans Blue dye leakage in mouse lungs treated with LPS for 2 days (n=10, *,P<0.01, unpairedT-test). (c) Graph showing the whole lung stiffness of LPS-treated lungs (n=8, *,P<0.05, unpairedT-test). (d) Graph showing LOX mRNA levels in LPS-treated lungs (n=10, *,P<0.01, unpairedT-test). (e) Graph showing LOX activity in mouse lungs treated with LPS (n=10, *,P<0.05, unpairedT-test). (f) Immunoblots showing LOX, LOXL1, LOXL2 and β-actin protein levels in mouse lungs treated with LPS. SeeSupplementary Fig. S5afor full-length blots. Immunoblots are showing representative results of three replica experiments. Error bars represent s.e.m. Figure 4: Lung vascular permeability in endotoxin-induced lung injury in vivo . ( a ) Immunofluorescence micrographs showing low MW fluorescently labelled dextran leakage (green) and blood vessel formation (CD31 staining; magenta) in LPS-treated mouse lung (for 2 days, bar, 10 μm). ( b ) Vascular permeability detected by Evans Blue dye leakage in mouse lungs treated with LPS for 2 days ( n =10, *, P <0.01, unpaired T -test). ( c ) Graph showing the whole lung stiffness of LPS-treated lungs ( n =8, *, P <0.05, unpaired T -test). ( d ) Graph showing LOX mRNA levels in LPS-treated lungs ( n =10, *, P <0.01, unpaired T -test). ( e ) Graph showing LOX activity in mouse lungs treated with LPS ( n =10, *, P <0.05, unpaired T -test). ( f ) Immunoblots showing LOX, LOXL1, LOXL2 and β-actin protein levels in mouse lungs treated with LPS. See Supplementary Fig. S5a for full-length blots. Immunoblots are showing representative results of three replica experiments. Error bars represent s.e.m. 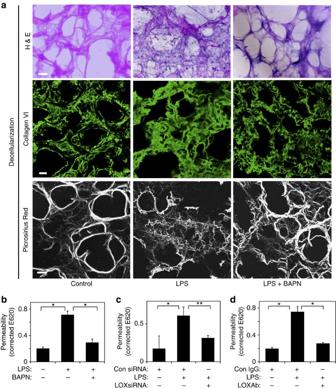Figure 5: ECM structure mediates lung vascular permeability in endotoxin-induced lung injuryin vivo. (a)Top, Light (H & E-stained) micrographs showing ECM structure of decellularized lung treated with LPS or in combination with BAPN (bar, 3 μm).Middle, Immunofluorescence micrographs showing the collagen VI distribution in the lung treated with LPS or in combination with BAPN after decellularization (bar, 4 μm).Bottom, birefringence (Picrosirius Red-stained) micrographs showing collagen structure in the lung treated with LPS or in combination with BAPN after decellularization (bar, 3 μm). (b–d) Graphs showing endothelial permeability detected by Evans Blue dye leakage in the lungs treated with LPS in combination with (b) BAPN (n=8, *,P<0.01, unpairedT-test), (c) control siRNA (con siRNA) or LOX siRNA (n=8, *,P<0.01, **,P<0.05, unpairedT-test), or (d) control IgG (con IgG) or LOX inhibitory Ab (n=6, *,P<0.01, unpairedT-test). All error bars are s.e.m. Full size image Figure 5: ECM structure mediates lung vascular permeability in endotoxin-induced lung injury in vivo . ( a ) Top , Light (H & E-stained) micrographs showing ECM structure of decellularized lung treated with LPS or in combination with BAPN (bar, 3 μm). Middle , Immunofluorescence micrographs showing the collagen VI distribution in the lung treated with LPS or in combination with BAPN after decellularization (bar, 4 μm). Bottom , birefringence (Picrosirius Red-stained) micrographs showing collagen structure in the lung treated with LPS or in combination with BAPN after decellularization (bar, 3 μm). ( b – d ) Graphs showing endothelial permeability detected by Evans Blue dye leakage in the lungs treated with LPS in combination with ( b ) BAPN ( n =8, *, P <0.01, unpaired T -test), ( c ) control siRNA (con siRNA) or LOX siRNA ( n =8, *, P <0.01, **, P <0.05, unpaired T -test), or ( d ) control IgG (con IgG) or LOX inhibitory Ab ( n =6, *, P <0.01, unpaired T -test). All error bars are s.e.m. Full size image Increased vascular permeability and pulmonary oedema are prominent features of acute lung injury and ARDS, which are commonly assumed to be controlled by levels of critical soluble cytokines, such as VEGF and TNFα ( [7] , [8] , [11] , [12] ). Here we show that changes of ECM structure and mechanics have an equally important role in control of vascular permeability and endotoxin-induced pulmonary oedema. Strikingly, the potent effects of endotoxin on pulmonary vascular permeability can be prevented by manipulating ECM structure, and hence, this mechanical control pathway could potentially lead to new approaches to clinical therapy in the future, in addition to providing greater insight into how changes in pulmonary microvascular structure influence organ pathophysiology. Changes in LOX activity levels that alter tissue structure and ECM mechanics contribute to many pathological processes that are characterized by abnormal vascular permeability, including fibrotic disorders [33] , [39] and cancer progression [13] , [37] , as well as cardiovascular diseases [20] , [40] , [41] . Our results show that ECM mechanics need to be regulated tightly to maintain optimal cell–cell junctional integrity and pulmonary vascular function in normal lung. Specifically, using various LOX inhibitors (BAPN, LOX-specific inhibitory Ab and LOX siRNA), as well as LOX overexpression, we found that changes in ECM structural crosslinking and rigidity that deviate from the normal range (either too rigid or too flexible) result in increased vascular permeability in vivo , just as altering ECM mechanics does in vitro . LOX manipulation altered lung stiffness between 1,000 and 2,500 Pa, which resulted in changes in vascular permeability in the lung in vivo ( Fig. 2 ). In contrast, while we observed a similar qualitative permeability response to changes in stiffness within endothelial cells cultured on ECM gels, the absolute values of stiffness were very different (cell–cell junctions were disrupted on ECM gels with 150 Pa or 35,000 Pa). This is likely because of difference in the measurement tools we utilized (rheology of cultured gels versus tensile loading of whole lung sections), which can produce different values of mechanical properties based on the area to which force is applied [42] . In addition, our in vitro studies employed only endothelial cells cultured on top of gels composed of one type of ECM component, whereas whole lung contains various cell types grown within three-dimensional ECMs composed of a complex array of insoluble ECM components and bound growth factors. In addition, lung epithelial and stromal cells secrete soluble factors and ECM proteins differently in response to changes in ECM mechanics, which might feedback to further alter ECM remodel and mechanics; changes in permeability in vivo also can result in fibrin deposition, which can further alter ECM stiffness. In any case, our studies show that endothelial cells exhibit a similar qualitative vascular permeability response to changes in mechanics in vitro and in vivo , much as we previously showed for their angiogenic response to alterations in ECM stiffness [15] . These studies show that ECM mechanics and structural changes need to be regulated carefully to maintain optimal pulmonary vascular function in the lung in vivo , just as we observed with cultured endothelial cells in vitro. Our studies have shown that ECM structure and elasticity control vascular permeability by altering formation of both VE-cadherin-containing adherens junctions and tight junctions [43] . The mechanism by which stiffness influences junctional integrity remains unclear; however, the localization of VE-cadherin is changed in a stiffness-dependent manner, with more VE-cadherin being present in the cytoplasm on more flexible substrates. One possible mechanism of control might involve the small GTPases, Rho and Rac, because ECM stiffness [44] and mechanical forces [45] , [46] control their activities, and Rho and Rac have been shown to regulate VE-cadherin localization and cell–cell junctional integrity [47] . As LOX can alter ECM structure in multiple ways through changing the expression or activities of various chemical factors that influence ECM metabolism (for example, transforming growth factor-β, MCP1 and so on) [48] , [49] , it is possible that ECM components other than collagens and elastins also contribute to the effects we observed. LOX inhibition also can render collagen more susceptible to degradation [50] ; however, we could not detect any change in collagen protein levels or degradation (measured by quantitating hydroxyproline levels) in BAPN-treated mice. On the other hand, past studies have shown that even a partial inhibition of collagen crosslinking results in changes in aortic wall stiffness [51] , [52] . BAPN treatment appears to produce similar changes of ECM structure and mechanics in the lung via induction of partial inhibition of collagen crosslinking, and thereby increases pulmonary vascular permeability in our system. LOX can increase production of reactive oxygen species, such as hydrogen peroxide, which can increase vascular permeability [53] . It is also possible that the collagen crosslinking modulating agents we used could produce similar effects by inducing an inflammatory cascade. However, these agents did not change the levels of inflammatory cytokines in the lung. Our finding that altering the stiffness of synthetic ECMs produces similar effects on junctional integrity and vascular permeability in vitro suggests that the effects of these agents on ECM mechanics represent the key control point for vascular barrier control. Our results clearly show that these agents, even in a short treatment (2 weeks of BAPN treatment and 1 week with LOX DNA/siRNA), changed collagen structure, fibre alignment and thickness. Therefore, these treatments affect lung vascular endothelial cell–cell junctional integrity at least partly by inhibiting collagen crosslinking. Mouse lungs treated with endotoxin LPS that exhibited greatly enhanced vascular permeability were much stiffer than non-treated lungs, suggesting that endotoxin might increase lung vascular leakage by altering ECM mechanics. However, leaky vessels might also release serum components that could, in turn, alter ECM structure; thus, this may involve a complex feedback loop in vivo . LPS rapidly enhances permeability and leukocyte extravasation, while ECM stiffness-mediated effects are more long term. Nevertheless, there is clear interplay between these chemical and structural changes in LPS-treated lungs because LOX inhibition restored the ability of LPS to increase vessel permeability. The variations in lung stiffness we measured may not reflect microscale changes in ECM elasticity, and thus, it is difficult to relate local changes in ECM mechanics to specific variations in vascular permeability within distinct regions of the lung. Nevertheless, taken together, these data suggest that ECM mechanics represents a previously unrecognized control point for vascular permeability control. In summary, these results demonstrate a novel mechanism for control of vascular permeability in which endothelial barrier function is regulated by changes in ECM mechanics mediated by LOX. This pathway also mediates the effects of endotoxin LPS on vascular leakage and pulmonary oedema, which can be prevented by modulating LOX activity. LOX activity and resulting changes of ECM structure could, therefore, represent novel therapeutic targets for control of pulmonary oedema, ARDS (for example, induced by sepsis), and a range of other diseases caused by abnormal vascular permeability. Materials Anti-CD31, and -VE-cadherin monoclonal antibodies (1:100 for staining) were from Transduction laboratory (Lexington, KY). Anti-collagen I, III, IV, VI, LOX, LOXL1 and LOXL2 polyclonal antibodies (1:100 for staining and 1:1 000 for immunoblotting) were from Abcam. Anti-ZO1 polyclonal Ab (1:100 for staining) was from Invitrogen. Anti-β-actin monoclonal Ab (1:1 000 for immunoblotting) was from Sigma. Anti-GAPDH Ab (1:5 000 for immunoblotting) was from Millipore. LOX-specific polyclonal inhibitory Ab was raised against the synthetic peptide of human/mouse LOX (EDTSCDYGYHRRFA) (Genscript, Piscataway, NJ) [13] , [36] , [37] . Mice treated with this LOX Ab exhibit reduced LOX activity and display significant decreases in LOX-mediated collagen crosslinking, as well as less linear collagen fibrils [13] , [36] . LPS and BAPN were from Sigma. L-HMVE cells (Lonza, Walkersville, MD) were cultured in EBM-2 (Cambrex) supplemented with 5% fetal bovine serum and growth factors according to the manufacturer’s instructions [3] . Plasmid construction and gene knockdown The full-length LOX plasmid was from Open Biosystems (Huntsville, AL) and subcloned into pOC mammalian expression vector. We used pOC vector as a control. Gene knockdown was performed using the RNA interference technique [15] . siRNA for mouse LOX was 5′-CAACGGGCAGGUGUUCAG-3′ and 5′-CUGAACACCUGCCCGUUG-3′ ( [54] ). As a control, siRNA duplex with irrelevant sequence (QIAGEN) was used. Biochemical Methods LOX activity in the serum and lung homogenate was measured using LOX activity assay kit (ABD Bioquest, CA) in which LOX substrate that releases hydrogen peroxide was detected [13] , [37] , [55] . Hydroxyproline in lung tissue or serum was measured using Hydroxyproline assay kit (Biovision, Milpitas, CA) [27] . The levels of IL-1 and TNF-α in the lung homogenate were measured by enzyme-linked immunosorbent assay (ELISA) (R&D systems). Molecular biological methods Quantitative reverse transcription (qRT)–PCR was performed with the Quantitect SYBR Green RT–PCR kit (QIAGEN) using ABI 7300 real time PCR system (Applied Biosystems, Foster City, CA). Cyclophilin controlled for overall complementary DNA content. The primers used for mouse cyclophilin were forward; 5′-CAGACGCCACTGTCGCTTT-3′, reverse; 5′-TGTCTTTGGAACTTTGTCTGCAA-3′ [15] . The primers for mouse LOX were forward; 5′-TCTTCTGCTGCGTGACAACC-3′, reverse; 5′-GAGAAACCAGCTTGGAACCAG-3′. Cell analysis methods L-HMVE cell monolayer junction formation was analysed using immunohistochemistry with VE-cadherin Ab staining [15] . Flexible polyacrylamide gel culture substrates were prepared using mixture of the acrylamide and the bis-acrylamide [15] and coated with fibronectin (1 μg cm −2 ), collagen I and -IV (1 μg cm −2 ). Substrate flexibility was controlled by varying the acrylamide (2–4%) and the bis-acrylamide (0.1–0.5%) concentration; the Young’s modulus (stiffness) was determined using rheology [56] . L-HMVE cells were cultured for 12 h on the gels and immunostaining was performed and analysed using confocal Leica SP2 microscope [15] . The integrity of the L-HMVE cell monolayer was evaluated by measuring TEER. In Transwell cultures, TEER was measured using a Millicell ERS meter (Millipore, Bedford, MA) coupled to a chopstick-like electrode, and TEER values ( U × cm 2 ) were determined by subtracting the baseline resistance value measured in the absence of cells and then multiplying the remaining ‘specific’ resistance value ( U ) times the cell culture surface area (cm 2 ) ( [57] ). In Vivo Pulmonary Permeability Assay The in vivo animal study was carried out in strict accordance with the recommendations in the Guide for the Care and Use of Laboratory Animals of the National Institutes of Health. All animal studies were reviewed and approved by the Animal Care and Use Committee of Boston Children’s Hospital. Mice (6–10 weeks old, CD1 strain, female) were treated with LPS (100 μg, intraperitoneally) and lung permeability was assessed 2 days after injection [3] . For gene knockdown or gene overexpression, delivery of siRNA and DNA into mice was performed using retro-orbital injection of the mixture with jet PEI (PolyPlus) or Exgen (Fermentas) per the manufacturer’s instructions, respectively [3] , [23] , [24] , [58] . Control DNA (vector only) and siRNA with irrelevant sequence were used as controls; these delivery methods have been shown not to elevate the serum levels of major pro-inflammatory cytokines (for example, TNF-α, IL-6 and so on) [59] . Gene knockdown or overexpression in the lung (2 days later) was confirmed by measuring mRNA and/or protein levels using qRT–PCR and IB, respectively. The lung permeability was measured using Evans Blue dye or low MW fluorescently labelled dextran (MW 4000, Sigma) leakage [3] . Evans blue dye was extracted from the lung by incubation with formamide (70 °C for 24 h) and the concentration of Evans blue was estimated by dual-wavelength spectrophotometer (620 nm and 740 nm). Mice were treated with BAPN (3 mg kg −1 , drinking water) for 14 days [13] . We also treated mice with LOX function-blocking polyclonal Ab (3 mg kg −1 ) ( [13] , [36] ), LOX DNA or LOX siRNA (10μg per mouse) injected intravenously (retro-orbital injection) twice per week. We treated the mice with LPS for the last 2 days. For decellularization of lung, we perfused the lung with decellularization buffer (0.5% SDS/PBS) for 1 h and cryosectioned it and analysed by Haematoxylin and eosin (H & E) staining and immunohistochemistry [25] , [26] . We confirmed that the collagen immunofluorescence staining we observed is specific and not due to autofluorescence using a secondary only control (rabbit IgG secondary used for all anti-collagen antibodies) ( Supplementary Fig. S2b ). For analysis of collagen structure, we used picrosirius red staining [30] and observed the structure using birefringence microscope (Abrio imaging system, CRI, MA) [30] . For TEM, small pieces (1–2 mm cubes) of lung tissue were fixed with 2.5% glutaraldehyde and 2% paraformaldehyde in 0.1 M sodium cacodylate buffer (pH 7.4) for at least 2 h at RT, washed in 0.1 M cacodylate buffer and postfixed with 1% Osmium tetroxide (OsO4)/1.5% Potassium ferrocyanide (K 4 FeCN 6 ) for 1 h, washed in water and incubated in 1% aqueous uranyl acetate for 1 h followed by washes in water and subsequent dehydration in grades of alcohol. The samples were then put in propyleneoxide for 1 h and infiltrated ON in a 1:1 mixture of propyleneoxide and TAAB Epon (Marivac Canada Inc. St Laurent, Canada). The samples were then embedded in TAAB Epon and polymerized at 60 °C for 48 h. Ultrathin sections (about 60 nm) were cut on a Reichert Ultracut-S microtome, picked up on to copper grids stained with lead citrate and examined in a JEOL 1400 TEM microscope or a TecnaiG 2 Spirit BioTWIN. BAL was performed by instilling 0.9% NaCl in two separate 0.5 ml aliquots. The fluid was recovered by gentle suction and placed on ice for immediate processing. An aliquot of the BAL fluid was processed immediately for differential cell counts performed on cytospin preparations stained with modified Wright-Giemsa stain (Diff-Quik; American Scientific Products, McGaw Park, IL). Measurement of lung stiffness We trimmed and made cylindrical lung tissue sections using a sharp knife that included peripheral and central portions of the left lobe. The stiffness of mouse lung tissues was evaluated by determining Young’s Modulus (E) under tensile loading [31] , [32] (Mach-1; Biomomentum, Canada). Tissues were attached to the base and probe using polyacrylamide glue and stretched until complete breakage of the tissue. The Young’s Modulus was derived from the slope of a standard stress–strain curve using data within the first 10% of the maximum strain. Statistical analysis All statistical data was analysed using GraphPad Prism V5.0. Error bars (s.e.m.) and P -values were determined from the results of at least three independent in vitro experiments and at least two independent in vivo experiments. The unpaired T -test was used for analysis of statistical significance. How to cite this article: Mammoto, A. et al . Control of lung vascular permeability and endotoxin-induced pulmonary oedema by changes in extracellular matrix mechanics. Nat. Commun. 4:1759 doi: 10.1038/ncomms2774 (2013).